Loss of flight promotes beetle diversification The evolution of flight is a key innovation that may enable the extreme diversification of insects. Nonetheless, many species-rich, winged insect groups contain flightless lineages. The loss of flight may promote allopatric differentiation due to limited dispersal power and may result in a high speciation rate in the flightless lineage. Here we show that loss of flight accelerates allopatric speciation using carrion beetles (Coleoptera: Silphidae). We demonstrate that flightless species retain higher genetic differentiation among populations and comprise a higher number of genetically distinct lineages than flight-capable species, and that the speciation rate with the flightless state is twice that with the flight-capable state. Moreover, a meta-analysis of 51 beetle species from 15 families reveals higher genetic differentiation among populations in flightless compared with flight-capable species. In beetles, which represent almost one-fourth of all described species, repeated evolution of flightlessness may have contributed to their steady diversification since the Mesozoic era. Insects are an extremely species-rich group with about 930,000 species [1] . One of the most important events in insect evolutionary history is the acquisition of flight, which occurred approximately 400 million years ago [2] . Flight ability facilitates the search and colonization of distant habitats, wide dispersal and the ability to find mates and food [2] , [3] , [4] . The evolution of flight is believed to have led largely to the diversification of insects through the exploitation of novel habitats and niches [1] , [2] , [5] . However, despite the advantages, many insect species of various lineages have lost their ability to fly [5] , [6] , [7] . Flightless species account for 10% of insect species diversity [5] , and species that are winged, but flightless due to the lack of flight muscles, are also expected to occur. The evolutionary loss of flight is attributed to the energetic cost associated with the maintenance of flight apparatuses, relative to other organs essential for survival and reproduction [8] , [9] , [10] . Low dispersal ability of flightless species leads to a low rate in gene flow, and as a consequence, differentiation among populations occurs [11] , [12] . Lower levels of dispersal result in higher rates of allopatric speciation [13] , [14] . Thus, the loss of flight in various lineages might be an important factor contributing to current insect diversity. Coleoptera comprises approximately 40% (350,000 species) of all insects, despite having evolved relatively recently among the insect orders [1] , [15] . Approximately 10% of the Coleoptera species are wingless [5] , although marked variations exist in flight ability among lineages. To test our hypothesis that the loss of flight promotes allopatric speciation and leads to higher species richness, we addressed, in detail, the causal relationship between flight loss and diversification using carrion beetles (Coleoptera: Silphidae) as a model system, two lineages of which (in the subfamily Silphinae) lost their flight ability due to evolutionary shifts in feeding habit [16] . We compared the geographical differentiation patterns and flight abilities of eight silphine species that are widely distributed throughout the Japanese archipelago, using population genetic approaches. We considered five species with flight muscles, two without flight muscles and one with flight muscle dimorphism [16] , [17] ( Supplementary Figure S1 ). The wide latitudinal range and complex topology of the Japanese archipelago have resulted in complicated distribution patterns of organisms, which provides an important resource for testing the effects of dispersal ability on allopatric speciation. We also conducted a meta-analysis of the genetic differentiation pattern among geographical populations of various beetle species to examine whether flight loss commonly promotes allopatric differentiation in Coleoptera. Flight ability and genetic differentiation To show that flightlessness promotes genetic differentiation among populations, we first performed an analysis of molecular variance (AMOVA) using 842 bp of the mitochondrial COI-II gene (novel accession codes AB606431 to AB606504, AB606597 to AB606661, Supplementary Table S1 ). 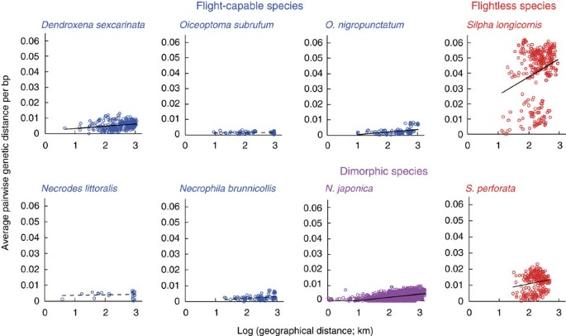Figure 1: Relationship between geographical and genetic distance in each species. Genetic distance is the average pairwise distance per base pair of theCOI-IIgene. Sample size (n), Mantel test (P-value) and slope of regression (b):Dendroxena sexcarinata,n=300,P<0.001,b=0.00062;Oiceoptoma subrufum,n=55,P=0.538,b=–0.00001;O. nigropunctatum,n=105,P=0.014,b=0.00075;Necrodes littoralis,n=21,P=0.197,b=0.00013;Necrophila brunnicollis,n=91,P=0.069,b=0.00049;N. japonica,n=3,655,P<0.001,b=0.00087;Silpha longicornis,n=325,P<0.001,b=0.00513;S. perforata,n=231,P=0.037,b=0.00165. In flight-capable species, the variance within populations explained most of the molecular variance (within populations: >93.5%; among populations: <6.5%), whereas the variance among populations explained most of the molecular variance in flightless species (within populations: 3.0 and 29.9%; among populations: 70.1 and 97.0%; Table 1 ). The species with flight muscle dimorphism showed an intermediate pattern between flight-capable and flightless species. Differentiation among populations was significant in flightless and dimorphic species. All species, except for three flight-capable species, showed significant isolation by geographical distance patterns in pairwise genetic distance for the COI-II gene ( Figure 1 ). The genetic differentiation was higher in flightless species than flight-capable species, suggesting that restricted gene flow due to flight loss resulted in higher genetic divergence at the same geographical distances. Table 1 Molecular variance and the number of potential species for the COI-II gene. Full size table Figure 1: Relationship between geographical and genetic distance in each species. Genetic distance is the average pairwise distance per base pair of the COI-II gene. Sample size ( n ), Mantel test ( P -value) and slope of regression ( b ): Dendroxena sexcarinata , n= 300, P <0.001, b= 0.00062; Oiceoptoma subrufum , n= 55, P= 0.538, b= –0.00001; O. nigropunctatum , n= 105, P= 0.014, b= 0.00075; Necrodes littoralis , n= 21, P= 0.197, b= 0.00013; Necrophila brunnicollis , n= 91, P= 0.069, b= 0.00049; N. japonica , n= 3,655, P <0.001, b= 0.00087; Silpha longicornis , n= 325, P <0.001, b= 0.00513; S. perforata , n= 231, P= 0.037, b= 0.00165. Full size image We also performed AMOVAs using two nuclear gene sequences, a 398-bp region of the phosphoenolpyruvate carboxykinase gene ( PepCK , novel codes AB668599 to AB668608, and AB668621 to AB668771, Supplementary Table S2 ) and a 386-bp region of the wingless gene ( Wg ; novel codes AB668609 to AB668620, and AB668772 to AB668939, Supplementary Table S2 ). 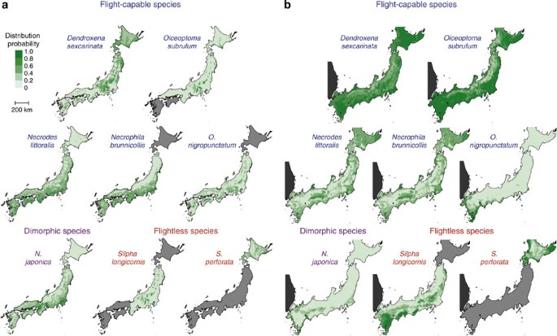Figure 2: Estimated potential distribution area for each species. (a) Potential distribution area at present. Pale gray areas represent regions where the species was assumed to be absent.Necrodes littoralis,Necrophila brunnicollis,N. japonicaandSilpha perforataoccur continuously in lowland areas, whereas the others (Dendroxena sexcarinata,Oiceoptoma subrufum,O. nigropunctatumandSilpha longicornis) are discontinuous in mountainous areas. (b) Potential distribution area during the Last Glacial Maximum (20,000 years ago). The dark gray area is a part of the East Asian mainland excluded from the estimated distribution area. The distribution areas of the montane species were more continuously distributed. The variances of these two nuclear genes were much lower than that of the COI-II gene, but the patterns in sequence divergence of these nuclear genes among species were largely consistent with that of the COI-II gene ( Table 2 ). Flightless and flight-dimorphic species showed higher genetic differentiations among populations compared with flight-capable species. The PepCK gene sequence of the flightless species Silpha perforata showed almost no differentiation. This species is a much more recent colonizer in Japan compared with another flightless species, S. longicornis [18] , and showed lower divergence than S. longicornis in all gene sequences. Table 2 Molecular variances for the PepCK and Wg genes. Full size table Effects of flight ability and habitat on genetic differentiation Discontinuity in distribution area can also contribute to differentiation among populations [19] , [20] . We estimated the distribution areas of each species from climatic variables to elucidate the relationship between the discontinuity of the potential distribution area and genetic differentiation. We also estimated the potential distribution areas during the Last Glacial Maximum (LGM; about 20,000 years ago), based on climatic variables reconstructed following previous studies [21] , [22] . The present and past distribution areas showed opposite patterns for each species because of climate change, indicating a long-term change in habitat discontinuity ( Figs 2a,b ; Supplementary Table S3 ). Note that flightlessness and habitat discontinuity were not necessarily linked. We calculated the index of discontinuity from the estimated distribution areas and examined the effect of flight loss and habitat discontinuity on genetic differentiation. The degree of molecular variance of the COI-II gene among populations was significantly higher in flightless than flight-capable species; present, but not past, habitat discontinuity also had a significant effect (generalized linear model (GLM) analysis, n= 8; flight ability: P <0.001; present distribution: P <0.001; past distribution: P =0.75; Supplementary Figure S2 ). Thus, the loss of flight has persistently accelerated genetic differentiation despite the changes in habitat distribution due to climate change. Figure 2: Estimated potential distribution area for each species. ( a ) Potential distribution area at present. Pale gray areas represent regions where the species was assumed to be absent. Necrodes littoralis , Necrophila brunnicollis , N. japonica and Silpha perforata occur continuously in lowland areas, whereas the others ( Dendroxena sexcarinata , Oiceoptoma subrufum , O. nigropunctatum and Silpha longicornis ) are discontinuous in mountainous areas. ( b ) Potential distribution area during the Last Glacial Maximum (20,000 years ago). The dark gray area is a part of the East Asian mainland excluded from the estimated distribution area. The distribution areas of the montane species were more continuously distributed. Full size image Effects of flight ability and habitat on speciation potential To compare the possibility of speciation between flight-capable and flightless species, we estimated the number of potential species (that is, genetically distinct units that can be treated as different demes) within each of the eight nominal species, based on the mitochondrial COI-II gene genealogy including all haplotypes ( Supplementary Figure S3 ). We used a generalized mixed Yule-coalescent (GMYC) approach [23] , [24] , which determines the threshold level to split species using a gene tree, and compared the number of potential species estimated from the GMYC approach for each nominal species between flight types. We simultaneously examined the effect of habitat persistence between the LGM and the present, because the habitat-type hypothesis predicts that persistent habitats favor organisms with low dispersal power [25] and that the speciation rate is higher for organisms associated with more persistent habitats [26] , [27] . We used changes in distribution probability between the LGM and the present as an index of habitat persistence. Under both the single- and multiple-threshold GMYC models, the number of potential species was significantly higher in flightless species than in flight-capable ones (GLM analysis; n= 8, P <0.001 in both models; Table 1 and Supplementary Figure S4 ), but was not related to habitat persistence (single model: P= 0.107, multiple model: P= 0.511). These results remained unchanged when GLM analyses were conducted with the numbers of potential species corrected for possible overestimation [28] (effect of flight ability: P <0.001 in both single and multiple models; effect of habitat persistence: P =0.122 and 0.072 in single and multiple models, respectively). Speciation rates in flight-capable and flightless lineages We compared the speciation and extinction rates between the flight-capable state and flightless state using a phylogenetic tree of Silphinae, constructed using two mitochondrial and three nuclear genes and the number of described species in each genus ( Supplementary Figure S5 ; potential species resulting from GMYC analysis are not considered here.). 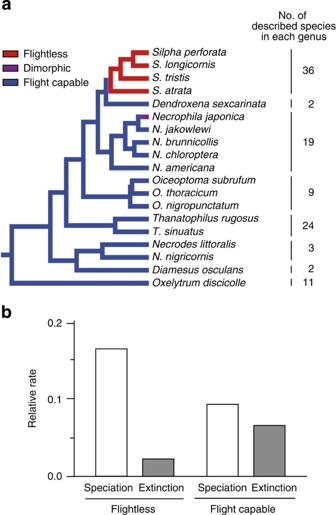Figure 3: Estimation of speciation rate for flightless and flight-capable states. (a) Phylogeny of Silphinae at the species level based onCOI-II,16S,28S,WgandPepckgene sequences. Number of described species48,49is assigned to each lineage. The numbers of described species in three genera that are not represented in this phylogenetic tree are included in the numbers of species of their sister genera (Supplementary Methods). (b) Speciation and extinction rate for flightless and flight-capable states in Silphinae. Speciation rate is significantly higher in flightless state than flight-capable state (likelihood ratio test; 2×log-likelihood difference=6.631,P<0.05). The speciation rate with the flightless state was twice that with the flight-capable state, whereas the extinction rate with the flightless state was lower than that with the flight-capable one ( Figure 3 ). The difference in speciation rates was significant in a likelihood ratio test (2×log-likelihood difference=6.631, P <0.05). Figure 3: Estimation of speciation rate for flightless and flight-capable states. ( a ) Phylogeny of Silphinae at the species level based on COI-II , 16S , 28S , Wg and Pepck gene sequences. Number of described species [48] , [49] is assigned to each lineage. The numbers of described species in three genera that are not represented in this phylogenetic tree are included in the numbers of species of their sister genera ( Supplementary Methods ). ( b ) Speciation and extinction rate for flightless and flight-capable states in Silphinae. Speciation rate is significantly higher in flightless state than flight-capable state (likelihood ratio test; 2×log-likelihood difference=6.631, P <0.05). Full size image Flight ability and genetic differentiation in Coleoptera To verify that the pattern shown in carrion beetles is common among different beetle families, we conducted a meta-analysis of the molecular variances among and within populations in COI-II and its adjacent gene regions, using data of 51 species from 15 coleopteran families ( Supplementary Table S4 ). As flightless species tended to have smaller geographical ranges than flight-capable species, we included the size of the sampling range as a variable to take into account its effect. 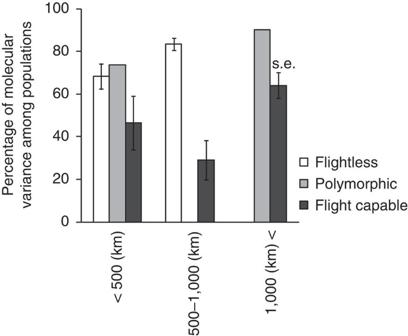Figure 4: Molecular variances among populations for flightless and flight-capable beetles. The percentages of molecular variances forCOI-IIand its adjacent DNA regions in flightless, polymorphic and flight-capable species are shown for each category of the geographical sampling range. Species with two or more flight morphs are categorized as polymorphic species. Graph shows mean±s.e. (standard error). The percentages of molecular variances among populations were significantly higher for flightless species than for flight-capable species (GLM analysis;n=48, flight ability:P<0.001, sampling range:P=0.021). The proportions of molecular variances among populations were significantly higher in flightless species than flight-capable species ( Figure 4 ; GLM analysis; n= 48, flight ability: P <0.001, sampling range: P =0.021), supporting the results shown in carrion beetles. Figure 4: Molecular variances among populations for flightless and flight-capable beetles. The percentages of molecular variances for COI-II and its adjacent DNA regions in flightless, polymorphic and flight-capable species are shown for each category of the geographical sampling range. Species with two or more flight morphs are categorized as polymorphic species. Graph shows mean±s.e. (standard error). The percentages of molecular variances among populations were significantly higher for flightless species than for flight-capable species (GLM analysis; n= 48, flight ability: P <0.001, sampling range: P =0.021). Full size image Our results demonstrate that the flightless species considered herein retained higher genetic differentiation among the populations than the flight-capable species, and that the diversification rate of the flightless lineage was higher than the flight-capable lineage. These data were obtained from a single group of beetles, Silphinae, but the results of our meta-analysis of the genetic differentiation patterns of various beetles suggested the generality of the causal relationship between flight loss and diversification. In four hyperdiverse insect orders (Hymenoptera, Lepidoptera, Diptera and Coleoptera), the loss-of-flight ability has occurred more frequently in families with more species, and this has been attributed to a large number of speciation events within these families, mostly due to chance [5] . In contrast, our results suggest that species richness may result from the loss of flight. The evolution of flight is thought to have led to the early diversification of insects [1] , [2] , [5] . However, after the insects had spread to different regions and occupied various habitats, allopatric speciation promoted by flight loss could have contributed to their increased diversity. As the evolution of flightlessness is often (but not necessarily) associated with the use of stable habitats [25] , habitat stability, rather than flight loss per se, may promote speciation [26] , [27] . In our analysis for Silphinae, however, the effect of habitat persistence on allopatric population divergence was not detected, whereas flight loss did have a significant effect. This result suggests that speciation rate is not strongly related to the habitat type in Silphinae, although additional analyses are needed. Importantly, the loss of flight in Silphinae is associated with an evolutionary switch in the feeding habit from vertebrate carcasses to invertebrates [16] . The loss-of-flight ability in different insect lineages could be due to diverse evolutionary changes in ecological traits such as food resources and habitat [5] . Therefore, our hypothesis of species diversification by loss of flight is not a subset of the habitat-type hypothesis of speciation. The speciation process through the loss of flight would be important, especially in Coleoptera. Our meta-analysis revealed that high molecular variance among the populations in flightless species compared with flight-capable ones is the common pattern among the different families of Coleoptera. One factor that has contributed to beetle diversity could be the adaptive radiation associated with the diversification of angiosperms in the Cretaceous [29] . However, a recent study revealed that the radiation of beetle families preceded the rise of angiosperms, and that different lineages have survived and continued to diverge ever since [30] . Flightless lineages are found throughout the beetle families and are especially common in ground beetles (Carabidae), which include about 40,000 species [1] , [9] . Although the proportion of wingless species in Carabidae is roughly estimated to be 20–25% [31] , a higher proportion would be flightless due to the lack of flight muscles, and hence, the overall proportion of flightless species should be higher. Therefore, loss of flight may be a common key event that contributes to the beetle diversification. Genetic differentiation among populations To compare the genetic differentiation pattern of the COI-II , Pepck and Wg genes among flight-capable, dimorphic and flightless species, we conducted AMOVA, using ARLEQUIN version 3.11 or 3.5 (ref. 32 ). We then compared the effect of isolation by geographical distance on the average pairwise genetic distance of the COI-II gene among flight-capable, dimorphic and flightless species. We conducted the Mantel test with 10,000 permutations using ARLEQUIN, to assess the relationship between the geographical distance and the genetic differentiation. In the Mantel test, the geographical distance was log 10 -transformed. Estimation of distribution areas To estimate species distributions at present and during the LGM, we determined the probability of occurrence in each 1-km mesh across Japan, using recent distribution records and 11 environmental variables obtained from the meteorological data for 1971–2000 by the program Maxent ver. 3.2.19 (ref. 33 ). The temperature during the LGM was assumed to be 11 °C lower than the present temperature, and the area was assumed to have experienced 1100/2100 times more precipitation than at present [21] . The maximum snow depth during the LGM was estimated from temperature and precipitation. We complemented the distribution probability at the LGM estimated from the Maxent program to include expanded land due to the regression of sea levels by the inverse-distance-weighted method using ArcGIS 9.3 (ESRI, Redlands, CA). Sea level at the LGM was assumed to be 120 m lower than at present [22] . Because of a limitation in the ArcGIS, the distribution probabilities at the LGM used in the following analyses were those calculated at a 3-km-mesh resolution. See also Supplementary Methods . Effects of flight ability and habitat on genetic differentiation We tested the effect of flight ability and habitat discontinuity on genetic differentiation by GLM analysis using JMP 6 software (SAS Institute Inc., Tokyo, Japan). We used the proportions of molecular variance of the COI-II gene among populations as the index of genetic differentiation. Flight ability was treated as an ordinal scale with three categories: flight-capable, dimorphic and flightless. We calculated the variance/mean ratio for the mesh data of the estimated distribution probability as the index of habitat discontinuity, where a higher value represents more discontinuity as in the index of aggregation [34] . To calculate this index, we pruned the southern, northern, eastern and the western edges of the mesh data for distribution probabilities of <20% to define the geographical areas of each species. The variance/mean ratio was then calculated from the remaining mesh data. We removed the non-distribution areas from the analyses. Normal distribution and identity link function were employed in the GLM analysis. We repeated the analyses, but changed the cutting threshold of the distribution probability from 20 to 40 or 60%. However, the results were similar for each percent probability (GLM analysis; 40%: flight ability: P <0.001, present distribution: P <0.001, past distribution: P =0.79; 60%: flight ability: P <0.001, present distribution: P <0.001, past distribution: P =0.68). Estimated number of potential species We constructed the maximum likelihood phylogeny of all COI-II haplotypes using the likelihood ratchet method and Phylogears2 ver. 2.0 (ref. 35 ) with TreeFinder, October version [36] . We conducted 100 replicates for the likelihood ratchet. Kakusan4 (refs 36 , 37 ) was used to determine appropriate models of sequence evolution by BIC4, and the GTR+G model was selected for the tree search. We converted the trees into ultrametric forms using the penalized likelihood method [38] implemented in r8s ver. 1.7 (ref. 39 ). We estimated the number of potential species within each of the eight nominal species from the converted tree using the GMYC approach [23] , [24] , which is implemented within the SPLITS package for R (available at http://r-forge.r-project.org/projects/splits/ ). In the GMYC method, the threshold time to separate species is determined from the tree. We conducted both the single-threshold model and the multiple-threshold model; the former determines one threshold level and the latter determines different threshold levels for distinct lineages. To examine the effects of flight ability and habitat persistence on the number of potential species, we conducted GLM analysis using the JMP 6 software (SAS Institute, Inc.). Flight ability was treated as an ordinal scale with three categories: flight-capable, dimorphic and flightless. As a variable representing habitat persistence during the last climatic change, we subtracted the distribution probabilities by a 3-km mesh at the LGM from those at present, and averaged the absolute differences across the distribution areas for each species. A Poisson distribution and logarithmic link function were used in the analysis. The use of GMYC approach in species delimitation is still controversial, especially for its accuracy in identifying actual demes [28] , [40] , [41] . GMYC analysis under incomplete geographical sampling overestimates the number of species, especially for the lineages with high rate of gene flow among the demes [28] . Thus, the results from GMYC analysis should be used with caution. As the number of potential species resulting from the GMYC analysis could be overestimated due to ignorance of the geographical distribution of the distinguished haplotype lineages, we corrected the number of potential species by combining multiple potential species, if any, that occurred in the same populations or a group of populations, and confirmed that all potential species after correction were geographically structured. Speciation rate in flight-capable and flightless lineages We constructed the phylogenetic tree of Silphinae using the COI-II , 16S , 28S , Wg and Pepck gene regions. The DNA sequences of the 16S , 28S , Wg and Pepck genes generated in a previous report [16] were used in this analysis. GenBank/DDBJ accession numbers of the COI-II region used for this analysis are given in Supplementary Table S1 . We used MUSCLE [42] in Mega5 Beta [43] with default parameter settings for the alignment. We constructed the maximum likelihood phylogeny using a likelihood ratchet method and Phylogears2 ver. 2.0 (ref. 35 ) with TreeFinder, October version [36] . We conducted 100 replicates for the likelihood ratchet. Kakusan4 (refs 36 , 37 ) was used to determine the appropriate models of sequence evolution by BIC4. The models for different genes (proportional model among regions and among codons; COI-II : GTR+Gamma; 16S : GTR+Gamma; 28S: GTR+Gamma; Pepck first codon: HKY85+Gamma; Pepck second codon: K80+Invariant; Pepck third codon: HKY85+Gamma; Wg first codon: JC69+Gamma; Wg second codon: JC69; Wg third codon: HKY85+Gamma) were used in the tree searches. We converted the trees into ultrametric forms, using the penalized likelihood method [38] implemented in r8s ver. 1.7 (ref. 39 ). We calculated the speciation and extinction rates using an ultrametric tree and compared the flight-capable and flightless states. These rates were estimated using a binary-state speciation and extinction model [44] , with the R package diversitree version 0.6 (ref. 45 ) via the Mesquite.R package [46] in Mesquite 2.74 (ref. 47 ). In this analysis, we used eight clades of Silphinae as the operational taxonomic units of the phylogenetic tree and assigned the number of described species in each clade (106 species in total based on Sikes [48] and Nishikawa et al . [49] : 36 flightless, 68 flight-capable and 2 unknown) and the incidences of three character states (flight-capable, flightless and unknown) in each clade. To investigate whether the difference in speciation rates between flight-capable and flightless states was significant, we conducted a likelihood ratio test [44] using the R package diversitree version 0.6 (ref. 45 ) via the Mesquite.R package [46] in Mesquite 2.74 (ref. 47 ). Log-likelihood values were obtained for models with no constraint on speciation rates and with the constraint of equal speciation rates for flightless and flight-capable states; in both models, the extinction rates were set as equal. The test statistic was 2×log-likelihood difference (6.631 in this analysis), with the 5% critical χ 2 =3.841 (df=1). See Supplementary Methods . Flight ability and genetic differentiation in Coleoptera We collected the data on genetic differentiation from published papers describing the proportion of molecular variance among and within populations in COI-II and its adjacent regions in beetles ( Supplementary Table S4 ). Flight ability was treated as an ordinal scale with three categories: flight-capable, polymorphic and flightless. The sampling range was also included as an ordinal scale with three categories: <500 km, 500–1,000 km and >1,000 km. We conducted GLM analysis using the JMP 6 software (SAS Institute, Inc.). If the molecular variance among populations was further divided into the variance among regional groups and the variance among populations within regional groups, we used the combined value of these variances as the variance among populations. Accession codes. The novel sequence data have been deposited in the GenBank database under accession codes AB606431 to AB606504 , AB606597 to AB606661 for COI-II ; AB668599 to AB668608 , and AB668621 to AB668771 for pepCK ; and AB668609 to AB668620 , and AB668772 to AB668939 for Wg . How to cite this article: Ikeda, H. et al . Loss of flight promotes beetle diversification. Nat. Commun. 3:648 doi: 10.1038/ncomms1659 (2012).